Anomalous piezoelectricity in two-dimensional graphene nitride nanosheets Piezoelectricity is a unique property of materials that permits the conversion of mechanical stimuli into electrical and vice versa. On the basis of crystal symmetry considerations, pristine carbon nitride (C 3 N 4 ) in its various forms is non-piezoelectric. Here we find clear evidence via piezoresponse force microscopy and quantum mechanical calculations that both atomically thin and layered graphitic carbon nitride, or graphene nitride, nanosheets exhibit anomalous piezoelectricity. Insights from ab inito calculations indicate that the emergence of piezoelectricity in this material is due to the fact that a stable phase of graphene nitride nanosheet is riddled with regularly spaced triangular holes. These non-centrosymmetric pores, and the universal presence of flexoelectricity in all dielectrics, lead to the manifestation of the apparent and experimentally verified piezoelectric response. Quantitatively, an e 11 piezoelectric coefficient of 0.758 C m −2 is predicted for C 3 N 4 superlattice, significantly larger than that of the commonly compared α-quartz. Availability of atomically thin piezoelectric materials are expected to have numerous applications in the area of nanoelectromechanical systems, which include stretchable smart electronics [1] , skins [2] , switches [3] and many types of sensors [4] , [5] , [6] , among others. Currently, boron nitride nanosheets appear to be the only material system that fit this profile. Recent works suggest that, somewhat thicker—at three atomic layers—molybdenum disulphide and tungsten disulphide sheets are also piezoelectric [7] . Graphene, owing to both its exotic properties and abundant availability, is arguably the most well-understood two-dimensional (2D) material and with several emergent applications [2] , [3] , [4] , [5] , [6] , [8] . Unfortunately, graphene is inherently non-piezoelectric and (usually) conductive (exceptions being certain configurations of graphene nanoribbons). Apparent piezoelectricity can be realized, however, through an interplay between symmetry, nanoscale size-effects and flexoelectricity—a material property that arises from the energy cost of creating internal polarizations in the presence of strain gradients. Borne out of these concepts, our quantum mechanical calculations have suggested that adding nanoscale triangular-shaped holes to edge-terminated graphene nanoribbons will lead to apparent piezoelectric behaviour [9] . In this work, we provide the first experimental evidence of this assertion. Nanometer-scale triangular holes are extremely difficult to fabricate in dielectric functionalized graphene nanoribbons [10] , [11] . Accordingly, we choose an alternative 2D structure: graphene nitride (C 3 N 4 ) nanosheets, which are electrically non-conducting. In graphitic form, carbon nitride’s structure naturally possesses regularly distributed triangular nanopores [12] . A stark difference to nanopores in pure graphene is that carbon and nitrogen atoms at the pore edges of graphene nitride are fully saturated; hence they require no passivation by any functional groups. Resulting from such structural stability, a bottom-up production of graphene nitride may be realized more straightforwardly, compared with porous graphene. A fabrication technique conveyed in this article is liquid-phase exfoliation. Graphene nitride, which intrinsically exhibits nanoscale pore sizes in the range of 1–2 nm, can be manufactured using this technique [11] . Graphene nitride, a commercial material, derived from elementary chemical building blocks has already found applications in fields such as catalytic enhancement and gas filtering [13] , [14] . However, potential roles of this material for piezoelectric devices remain largely unexplored. Using a state-of-the-art piezoresponse force microscopy (PFM) and results from ab initio calculations, we show that 2D graphene nitride is indeed piezoelectric with the corresponding coefficient significantly greater than that of α-quartz, and hence a promising candidate for nano- and micro-electromechanical applications. Structure of graphene nitride Carbon nitride, C 3 N 4 , is predicted to exist in α, β, cubic, pseudo-cubic and 2D graphitic (g) forms [12] . The graphitic form of carbon nitride is known as graphene nitride, or g-C 3 N 4 . A single sheet of g-C 3 N 4 may be composed of an s-triazine or tri-s-triazine repetition ( Fig. 1a ), with the tri-s-triazine form being the more energetically stable of the two structures [12] . The tri-s-triazine sheet of g-C 3 N 4 naturally has non-centrosymmetric, triangular holes throughout its structure. Therefore it is expected that the in-plane, e 11 , component of the piezoelectric tensor will be non-zero, where the ê 1 direction is aligned with the triangular holes as shown by the compass in Fig. 1a . The preferred stacking method for g-C 3 N 4 is by using a repeat unit in the symmetry group ( Fig. 1b ) with 3.29 Å spacing between sheets [15] . The metastable structure of β-C 3 N 4 ( Fig. 1c,d ) also has the interesting property of being predicted to be harder than diamond [16] . However, unlike the graphitic structure, the β form is centrosymmetric and therefore is not expected to exhibit piezoelectricity. Further information on β-C 3 N 4 will be provided in the computational section to verify that the statements made so far are correct. 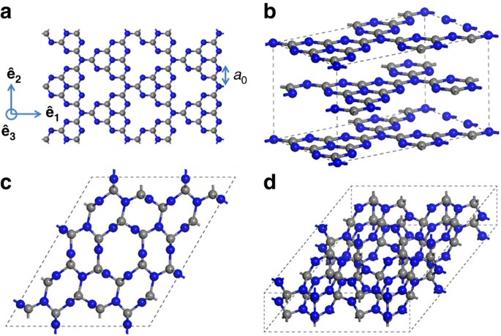Figure 1: Different forms of C3N4. Blue and grey spheres represent nitrogen and carbon atoms, respectively. (a) Single-sheet tri-s-triazine (g-C3N4). (b) Layered tri-s-triazine sheets. (c,d) β form shown from two perspectives to illustrate the three-dimensionality of the structure. Figure 1: Different forms of C 3 N 4 . Blue and grey spheres represent nitrogen and carbon atoms, respectively. ( a ) Single-sheet tri-s-triazine (g-C 3 N 4 ). ( b ) Layered tri-s-triazine sheets. ( c , d ) β form shown from two perspectives to illustrate the three-dimensionality of the structure. Full size image Fabrication of graphene nitride g-C 3 N 4 nanosheets were fabricated by liquid-phase exfoliation of commercially available g-C 3 N 4 powder (Carbodeon Ltd.) in 2-isopropanol (IPA). A silicon wafer was used for the main substrate; to increase the electrical conductivity of the substrate, a layer of gold was deposited onto the silicon before addition of the graphene nitride solution. In a typical fabrication, 30 mg of bulk g-C 3 N 4 was suspended in IPA to create yellow dispersion with a concentration of 3 mg ml −1 , and then the solution was sonicated at room temperature for the gradual exfoliation of bulk g-C 3 N 4 to nanosheets. This exfoliation process is similar to that reported for other layered materials (boron nitride, MoS 2 ) via the interaction of solvent molecules, which in turn is significantly influenced by the dispersive, polar and hydrogen-bonding solubility parameters of used solvents [17] . According to the Hansen solubility parameter theory, it is known that the layered materials can be successfully exfoliated when the enthalpy of mixing is minimized as the surface energies of flake and solvent match. The optimum surface energy of solvent is ~30 mJ m −2 , lower than that of van der Waals-bonded surfaces (~70 mJ m −2 ) [17] . Thus, IPA is a promising solvent for the exfoliation of bulk g-C 3 N 4 given its surface energy value (~40 mJ m −2 ). After sonication for 10 h, the dispersion was then centrifuged at 3,000 r.p.m. to remove aggregates, giving rise to a homogenous and light-yellow dispersion of g-C 3 N 4 nanosheets ( Fig. 2b ). As seen in Fig. 2a,b , the typical size of the fabricated nanosheet samples were around 800 nm in width, while their thicknesses, as measured by atomic force microscopy (AFM), were in the 1–2 nm range ( Fig. 2c ). The X-ray photoelectron spectroscopy survey spectra shown for the nanosheets in Fig. 2d confirm that the correct ratio of carbon to nitrogen atoms is achieved. Electron energy loss spectroscopy reveals that the fabricated sample possesses the expected sp 2 bonding between carbon and nitrogen atoms ( Fig. 2e ) [12] . 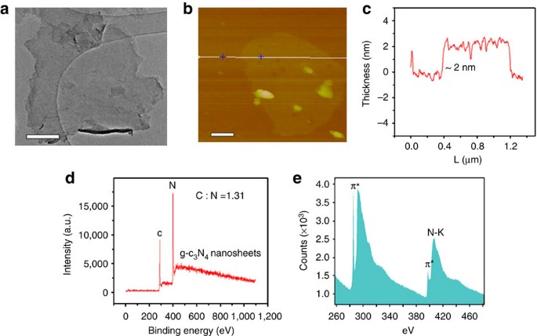Figure 2:Microscopy images of fabricated g-C3N4nanosheets. (a) Transmission electron microscopy (TEM) image of exfoliated g-C3N4nanosheets, scale bar, 200 nm. (b) Representative AFM image, scale bar, 200 nm, and (c) corresponding thickness analysis taken around the white line inbreveal an average thickness of about 2 nm for g-C3N4nanosheets. (d) X-ray photoelectron spectroscopy survey spectra of the exfoliated g-C3N4nanosheets, disclosing the atomic ratio of 1.31 between carbon and nitrogen. (e) Electron energy loss spectroscopy of g-C3N4nanosheets further reveals that both C and N have strongsp2bonding, as can be seen from the strong π* peaks. Figure 2: Microscopy images of fabricated g-C 3 N 4 nanosheets. ( a ) Transmission electron microscopy (TEM) image of exfoliated g-C 3 N 4 nanosheets, scale bar, 200 nm. ( b ) Representative AFM image, scale bar, 200 nm, and ( c ) corresponding thickness analysis taken around the white line in b reveal an average thickness of about 2 nm for g-C 3 N 4 nanosheets. ( d ) X-ray photoelectron spectroscopy survey spectra of the exfoliated g-C 3 N 4 nanosheets, disclosing the atomic ratio of 1.31 between carbon and nitrogen. ( e ) Electron energy loss spectroscopy of g-C 3 N 4 nanosheets further reveals that both C and N have strong sp 2 bonding, as can be seen from the strong π* peaks. Full size image PFM The piezoelectric property of the g-C 3 N 4 nanosheets is examined using PFM. For piezoelectric materials, an applied voltage will cause a measurable deflection of the cantilever [18] . The thickness of the fabricated nanosheets is in the order of only a couple nanometers, while the length and width can range from 500 nm to a few μm. For such dimensions, although it is easy to apply an in-plane bias by attaching electrodes to each end of the substrate, measuring the in-plane strain caused by the applied voltage is a daunting task. Accordingly, we have preferred the use of PFM. In order to verify the piezoelectricity of g-C 3 N 4 samples, a conductive scanning probe microscopy (SPM) tip is brought into contact with the sample, and an a.c. voltage is applied. The voltage is applied in the direction normal to the graphene nitride sheets ( ê 3 in Fig. 1a ), and is applied in such a manner that there are spherical symmetric components of the electric field along the in-plane axes ( ê 1 and ê 2 in Fig. 1a ), thus allowing for the measurement of different piezoelectric responses using the same method. If the sample is piezoelectric, local vibration underneath the SPM tip will be excited, and the resulting deflection of the cantilever can be recorded by a laser diode. In order to enhance the sensitivity of the measurement, the voltage is often applied near the cantilever-sample resonance, which magnifies the piezoelectric vibration by orders of magnitude. This vibration is indeed observed in g-C 3 N 4 samples, as shown in Fig. 3 . The vertical, out-of-plane, PFM response is shown in Fig. 3a under five different excitation voltages, which exhibit a clear resonant peak near 357 kHz. On the other hand, the lateral, in-plane, PFM response shown in Fig. 3c exhibits a resonant peak near 778 kHz. Here, lateral PFM response refers to cantilever twisting induced by in-plane piezoelectric shear strain, and the mode shapes for both the vertical and lateral PFM responses are found using the finite element method (FEM) simulation presented in the Methods section. By treating the cantilever-sample system as a damped harmonic oscillator, the quality factor can be fitted from the data, allowing us to determine the intrinsic piezoelectric response versus applied voltage, as shown in Fig. 3b,d . The amplitude shows a clear linear relationship with the excitation voltage for both vertical and lateral PFM, confirming the linear piezoelectricity of the sample. The effective vertical coefficient of the g-C 3 N 4 is estimated from the PFM data to be approximately 1 pm V −1 , while lateral deflection magnitude cannot be calibrated, and thus the lateral coefficient is not estimated. Nevertheless, the linear response is evident. 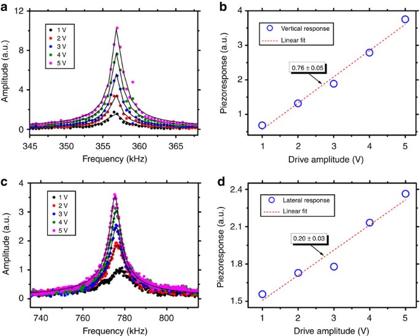Figure 3:Vertical and lateral PFM responses of g-C3N4across resonant frequency. (a,c) Resonant peaks for different applied voltages. (b,d) Linear correlation between the applied voltage and the amplitude of the displacement. Figure 3: Vertical and lateral PFM responses of g-C 3 N 4 across resonant frequency. ( a , c ) Resonant peaks for different applied voltages. ( b , d ) Linear correlation between the applied voltage and the amplitude of the displacement. Full size image To further examine the piezoelectricity, we probe a g-C 3 N 4 particle (containing many layers) on a conductive substrate, as shown in Fig. 4 . The topography mapping in Fig. 4a shows a clear particle approximately spherical in shape and 15 nm in height. The corrected PFM amplitude mapping in Fig. 4b shows large PFM response on the particle, but rather low response to its surroundings. The phase mapping in Fig. 4c shows uniform distribution of polarity in the particle. The mapping of resonant frequency is shown in Fig. 4d , wherein the contrast between g-C 3 N 4 particle and the conductive substrate is evident. g-C 3 N 4 exhibits a slightly smaller resonant frequency, suggesting that it is mechanically more compliant than its substrate. 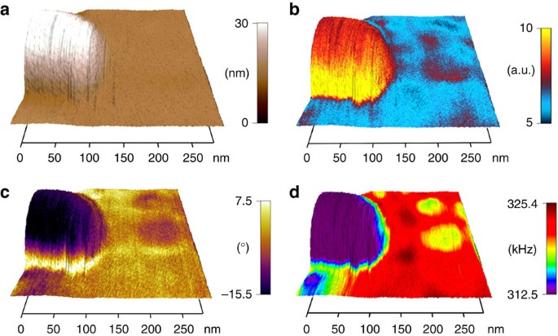Figure 4:PFM response of a g-C3N4particle on conductive substrate. (a) Topography; (b) corrected vertical PFM amplitude; (c) phase; and (d) resonant frequency. Figure 4: PFM response of a g-C 3 N 4 particle on conductive substrate. ( a ) Topography; ( b ) corrected vertical PFM amplitude; ( c ) phase; and ( d ) resonant frequency. Full size image Elucidation of the origin of anomalous piezoelectricity We believe that flexoelectricity, together with the presence of non-centrosymmetric holes, is the central reason that explains the emergence of apparent piezoelectricity in g-C 3 N 4 . Flexoelectricity is the development of polarization due to strain gradients. The polarization vector may be written as: Even in the absence of native piezoelectricity, polarization can be originated by non-uniform strains [9] . This phenomenon is illustrated in Fig. 5 . Consider a non-piezoelectric sheet without defects as displayed diagrammatically in Fig. 5a . Under a uniform stretch, the net polarization will be zero mainly because of the absence of intrinsic piezoelectricity. Now imagine a non-piezoelectric sheet with circular holes displayed in Fig. 5b . The same uniform stretch introduces the appearance of local polarization owing to flexoelectricity caused by strain gradients around the pore. However, there is zero piezoelectric response because the net average polarization is zero due to the symmetry of the circular hole. Finally, consider the case of non-centrosymmetric holes, for example, triangular-shaped ones in Fig. 5c . They will ensue a net average polarization under the action of a mechanical stretch (or compression). Consequently, a non-zero net piezoelectric response emerges. 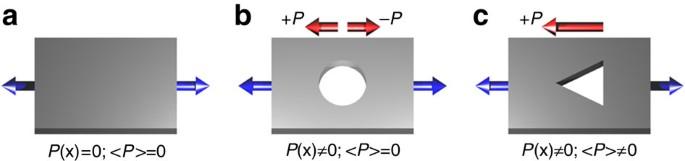Figure 5: Illustration of effects of nanopores on the polarization of a non-piezoelectric material under uniform stress. (a) A non-piezoelectric material with no pores exhibits no piezoelectric response; (b) with circular (centrosymmetric) pores, local polarization is non-zero while net polarization remains zero, and overall there is no apparent piezoelectric response; (c) with triangular (non-centrosymmetric) pores, a non-zero local and net polarization exist and the material possesses an apparent piezoelectricity. Figure 5: Illustration of effects of nanopores on the polarization of a non-piezoelectric material under uniform stress. ( a ) A non-piezoelectric material with no pores exhibits no piezoelectric response; ( b ) with circular (centrosymmetric) pores, local polarization is non-zero while net polarization remains zero, and overall there is no apparent piezoelectric response; ( c ) with triangular (non-centrosymmetric) pores, a non-zero local and net polarization exist and the material possesses an apparent piezoelectricity. Full size image From symmetry arguments, it is immediately clear that for a flat sheet, or even a stack of sheets, there should be only one independent non-zero component of the piezoelectric tensor (total of three non-zero components); that is the e 11 coefficient corresponding to in-plane polarization and strain measured in the same direction [19] . Using the difference in polarization, in the ê 1 direction (as shown in Fig. 1a ), components between the unstrained state and the strained state, the piezoelectric coefficient, e 11 , can be found from the simple relation obtained by differentiating equation (1) [19] as: The numerical values of the apparent piezoelectric coefficients of g-C 3 N 4 can be calculated from first principles. Here, all quantum calculations are based on the density functional theory (DFT) as implemented in the Quantum Espresso software and using ultrasoft pseudopotentials, C.pz-van_ak.UPF for carbon and N.pz-van_ak.UPF for nitrogen atoms, from the Quantum Espresso pseudopotential database [20] ( http://www.quantum-espresso.org/pseudopotentials ). To achieve the best efficiency, some of the key parameters were a priori optimized for the calculations. These parameters are shown in Table 1 , and include the lattice constant, a 0 , the spacing between sheets, c , the cutoff energy and the Monkhorst-Pack k -point grid for Brillouin zone integration. The lattice constant given is the distance between two like atoms, not the entire length of the unit cell. The parameters for the β form should not be directly compared with the graphitic single sheet and stacked structures owing to the different symmetry group. For the single sheet, a spacing of 4.28 Å is found to be sufficient to assure that there is no interaction between periodic images. Table 1 Parameters used for quantum calculations. Full size table The same procedure is applied to compute piezoelectric coefficients of the sheet, β, and stacked structures. The calculations are performed in an unstrained reference state and under various levels of strain up to 1%; the strain is applied in the ê 1 direction, as shown by the arrow in Fig. 1a . After applying the strain, the system is relaxed, while the box size is kept fixed, until the force on each atom is below 0.0019 Ry Å −1 . The polarization is then estimated using the Berry-phase method for both the unstrained and strained cases [21] , [22] . The computed change in polarization along with the predicted piezoelectric coefficient for each form of carbon nitride tested is shown in Table 2 , obtained from a least squares fit of the data. These results confirm the central notion that g-C 3 N 4 is piezoelectric, while β-C 3 N 4 , is not. The complete results of all calculations performed for the stacked configuration are shown in Fig. 6 , illustrating the expected linear piezoelectric response. Note that the piezoelectric coefficient is given per unit volume. Estimating a quantity per unit volume for an infinitely thin sheet is ill-defined. In order to directly compare all of the tested configurations, the difference in polarization between the strained and unstrained systems, ΔP 1 , is given in units such that it is independent of the volume used in the calculations. Therefore, the value of e 11 given for the single sheet in Table 2 is an ‘effective’ piezoelectric coefficient, that is, using the ratio of ΔP 1 to e 11 found for the stacked configuration. As seen from Table 2 , the piezoelectric coefficients of both stacked and single-layer g-C 3 N 4 are over four times greater than that of α-quartz. The full piezoelectric tensors for both the stacked and single-layer graphene nitride are provided in Supplementary Figs 1 and 2 , respectively. Comparing the ΔP 1 for each configuration shows that there is a very slight increase (~3%) in the piezoelectric properties of g-C 3 N 4 when multiple sheets are present. Table 2 Quantum calculation results. 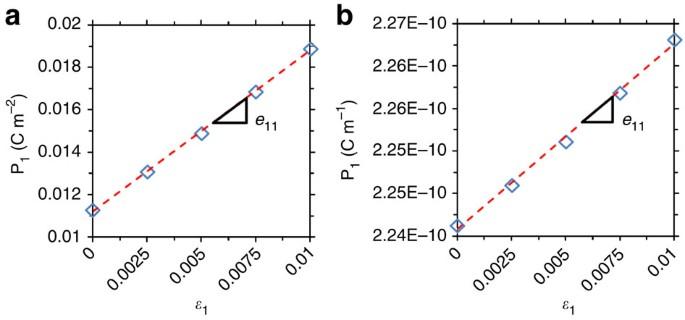Figure 6: Polarization versus strain curve for graphitic carbon nitride obtained from quantum mechanics calculations. A clear linear correlation is evident, and the slope, corresponding to the piezoelectric coefficient, is shown for (a) the stacked configuration in C m−2, (b) a single sheet in C m−1. Full size table Figure 6: Polarization versus strain curve for graphitic carbon nitride obtained from quantum mechanics calculations. A clear linear correlation is evident, and the slope, corresponding to the piezoelectric coefficient, is shown for ( a ) the stacked configuration in C m −2 , ( b ) a single sheet in C m −1 . Full size image The e 11 coefficient for the single sheet is also reported in C m −1 , the conventional units for 2D materials, in Table 3 . The result is compared with those of other 2D structures also found using DFT calculations. Graphitic carbon nitride sheets exhibit a greater piezoelectric response than hexagonal boron nitride (h-BN), but below that of molybdenum disulphide (MoS 2 ). The most comparable material, in terms of piezoelectric properties, is tungsten disulphide (WS 2 ), which possesses a slightly higher e 11 coeffiecient [7] . Table 3 Comparison of 2D piezoelectrics. Full size table The materials compared in Table 3 also exhibit a unique disadvantage when compared with g-C 3 N 4 —they lose their piezoelectric effect when >1 layer is present. Bulk forms of MoS 2 , h-BN or WS 2 are indeed centrosymmetric, owing to an antiparallel stacking sequence, and thus not piezoelectric [7] . However sheets of g-C 3 N 4 are not stacked in the same manner to form a bulk material and piezoelectricity is retained; the stacking sequence here is analogous to that of graphite [15] . Therefore, it is clear that the regularly placed triangular holes are indeed responsible for the apparent piezoelectric coupling found in graphene nitride. Without these holes, the material would be essentially the same as boron nitride, which loses its piezoelectricity when multiple layers are present. Regarding the experimental results, our current apparatus cannot fully measure the common e 11 piezoelectric coefficient to enable a direct comparison. However, the experimental results presented are sufficient to prove that graphitic carbon nitride is indeed piezoelectric, although the out-of-plane PFM measurements of effective e 33 coefficient do not directly match with both quantum mechanics results and crystal symmetry considerations where the e 33 coefficient is identically zero. This is not completely unexpected, since other piezoelectric coefficients contribute to out-of-plane deflection too. There are additional possible reasons for this discrepancy as well. As seen specifically from the AFM result in Fig. 2c , which depicts the thickness profile across g-C 3 N 4 nanosheets and the substrate, it is clear that the samples used in the PFM experiments are not perfectly flat. The departure from perfect flatness will lead the presence of non-zero out-of-plane polarization. Another possibility is that the fabrication of nanosheets resulted in non-uniform samples that are not aligned both along in-plane and out-of-plane directions; this is tentatively supported by the transmission electron microscopy and AFM images shown in Fig. 2a,b . Finally, the disagreement could also stem from the substrate itself. A lattice mismatch between the g-C 3 N 4 and the substrate may lead to an induced strain at the bottom of the sample, resulting in a possible out-of-plane polarization component. As an additional measure, FEM simulations have been employed, as explained in the methods section, to show that with the current PFM setup and predicted piezoelectric coefficients from DFT, an out-of-plane response can arise although the e 33 coefficient is zero. The FEM results, combined with the other possibilities, provide a rigorous link between the experimental data and the quantum mechanics calculations. In summary, we have experimentally shown that g-C 3 N 4 is piezoelectric and atomistically elucidated the mechanisms that lead to the emergence of this anomalous behaviour. The calculated e 11 piezoelectric coefficient of bulk g-C 3 N 4 is 0.758 C m −2 , significantly greater than that of α-quartz (0.171 C m −2 ), while the 2D coefficient is higher than that of other known atomically thin piezoelectrics such as h-BN. Higher piezoelectric response suggests that g-C 3 N 4 may be used where more sensitive electromechanical coupling is required. This makes g-C 3 N 4 , in either bulk or single-layer form, a promising candidate material for use in nanoelectromechanical systems requiring piezoelectric materials. The presence of piezoelectric coupling in the bulk phase also signifies that manufacturing a single-atomic layer material is not necessary for applications where minimal thickness is not a major constraint. PFM For PFM, the probe used is an ASYELEC-01 silicon probe with Ir reflex and tip coated. The nominal stiffness is 1.59 N m −1 , and the applied force is 152 nN. The applied electric field has a three-dimensional distribution, with both out-of-plane and in-plane components, such that the measured vibrations have multiple contributions from different piezoelectric tensor components. This allows us to test various piezoelectric coefficients with the same experimental setup. To verify that our PFM method will actually test the electromechanical coupling of a system, several control tests were performed using the same procedure as described in the paper. As a control, we measured the response of a plastic sample on a gold-coated silicon substrate as well as that of the gold coating itself. The vibrational responses of these controls, along with those measured on a C 3 N 4 sample on a gold-coated silicon substrate, are shown in Supplementary Fig. 3 (vertical PFM) and Supplementary Fig. 4 (lateral PFM). As expected, no clear resonance peak is observed in plastic since it possesses no piezoelectric properties. There is a peak observed for the bare gold coating, this can be attributed to electrostatic interactions. The g-C 3 N 4 sample shows clear peaks at the resonant frequencies. The samples are tested at frequencies near the resonant frequencies of the two different vibration modes of the cantilever. The frequency at 357 kHz corresponds to the first eigen mode of normal deflection, under vertical PFM, and the 778 kHz frequency is the eigen mode related to the twisting (shearing) of the cantilever, under lateral PFM. Finite element simulations for these two vibration modes have been carried out, as presented in the corresponding section. The comparison of the response versus voltage, between gold coating and g-C 3 N 4 is shown in Supplementary Fig. 5 . As we monitor the voltage versus amplitude, it becomes clear that the bare gold substrate does not exhibit a linear response that would be expected of a piezoelectric material. Therefore, although gold does show peaks at the resonant frequencies in Supplementary Figs 3 and 4 , evidently this is not due to any electromechanical coupling of the material. Meanwhile, our g-C 3 N 4 sample does show a linear increase in amplitude as the applied voltage is increased, typical of the characteristic of a piezoelectric material being tested in PFM. Differences in mechanical properties are demonstrated through changes in contact resonance. However, the primary contribution to contact resonant shift is changes in contact stiffness, although contact area variation can also be partially responsible, which can be minimized by maintaining constant contact force. In our experiment, through feedback control, the system kept a constant contact force while scanning through feedback control. We expect that different contact forces do not affect the response much. Finite element method simulations A finite element calculation using COMSOL is performed modelling the PFM setup to help elucidate the relationship between the experimental results and quantum calculations. The FEM model is able to show that with the predicted piezoelectric coefficients of g-C 3 N 4 from DFT calculation both a vertical, out-of-plane and a lateral, in-plane response can be resulted in PFM experiments, although e 33 and e 15 are zero. This is clear from Supplementary Fig. 6 , where the total displacement field in the sample underneath a charged SPM tip is shown, and both vertical and lateral displacements are observed. The dynamic responses of the cantilever excited by piezoelectric effect of g-C 3 N 4 are shown in Supplementary Fig. 7 (vertical PFM) and Supplementary Fig. 8 (lateral PFM), and we notice reasonable agreement on resonant frequencies for both vertical and lateral PFM between experiments and simulations. Quantum calculations The full piezoelectric tensors for both the single sheet and stacked configurations are given in Supplementary Figs 1 and 2 , respectively. On the basis of symmetry arguments for the class, there should be three non-zero components and only one independent component [19] . These three coefficients are related by the relations: This is supported by the results found using DFT as previously described. The results from the bulk and single-sheet configurations can be compared to verify that these results are correct. If the single-sheet coefficient is divided by the spacing between sheets in the stacked form to convert from a per area quantity to a per volume amount, the result should be the same as the ‘effective’ piezoelectric constant given for the single sheet in Table 2 . Following this previous statement, we obtain the result: Supplementary Figs 1 and 2 show that the relations given inequations (3) and (4) are correct. There are some slight differences that can be attributed to numerical error caused by using relatively low cutoff energies and less densely packed k -point grids to speed up the DFT calculations. All of the results are within a reasonable accuracy, so we find no need for further intensive calculations. Components suspected to be zero were also tested in order to verify that the symmetry arguments made earlier are correct. How to cite this article : Zelisko. M. et al. Anomalous piezoelectricity in two-dimensional graphene nitride nanosheets. Nat. Commun. 5:4284 doi: 10.1038/ncomms5284 (2014).